Geographic population structure analysis of worldwide human populations infers their biogeographical origins The search for a method that utilizes biological information to predict humans’ place of origin has occupied scientists for millennia. Over the past four decades, scientists have employed genetic data in an effort to achieve this goal but with limited success. While biogeographical algorithms using next-generation sequencing data have achieved an accuracy of 700 km in Europe, they were inaccurate elsewhere. Here we describe the Geographic Population Structure (GPS) algorithm and demonstrate its accuracy with three data sets using 40,000–130,000 SNPs. GPS placed 83% of worldwide individuals in their country of origin. Applied to over 200 Sardinians villagers, GPS placed a quarter of them in their villages and most of the rest within 50 km of their villages. GPS’s accuracy and power to infer the biogeography of worldwide individuals down to their country or, in some cases, village, of origin, underscores the promise of admixture-based methods for biogeography and has ramifications for genetic ancestry testing. The ability to identify the geographic origin of an individual using biological data, poses a formidable challenge in anthropology and genetics because of its complexity and potentially dangerous misinterpretations [1] . For instance, owing to the intrinsic nature of biological variation, it is difficult to say where one population stops and another starts by looking at the spatial distribution of a trait (for example, hair colour [2] ). Darwin acknowledged this problem, stating that ‘it may be doubted whether any character can be named which is distinctive of a race and is constant’ [3] . Yet, questions of biogeography and genetic diversity such as ‘why we are what we are where we are?’ have piqued human curiosity as far back as Herodotus of Halicarnassus, who has been called ‘the first anthropologist’ [4] . However, only in the past decade have researchers begun harnessing high-throughput genetic data to address them. The work of Cavalli-Sforza and other investigators [5] , [6] , [7] established a strong relationship between genetic and geographic distances in worldwide human populations, with major deviations explicable by admixture or extreme isolation [8] . These observations, stimulated the development of biogeographical methods. Accurate measurements of biogeography began at the cusp of the DNA sequencing era and have since been applied extensively to study genetic diversity and anthropology [9] , [10] , infer origin and ancestry [11] , [12] , map genes [13] , identify disease susceptibility markers [2] and correct for population stratification in disease studies [14] . Biogeographic applications currently employ principal component (PC)-based methods such as PC analysis (PCA), which was shown to be accurate within 700 km in Europe [11] , and the most recent Spatial Ancestry Analysis (SPA) [12] that explicitly models allele frequencies. Yet, estimated by the percentage of individuals correctly assigned to their country of origin, the accuracy of PCA and SPA is relatively low for Europeans (40±5 and 45±5%, respectively) and much lower for non-Europeans [12] . Such results suggest limitations with these approaches for biogeographical inference [12] , [15] , [16] , coupled with a possible limitation of commonly used genotyping arrays in capturing fine substructure [17] , [18] . As patterns of genetic diversity in human populations or admixture are frequently described as genome-based estimates of several ancestries that sum to 100% (refs 19 , 20 , 21 ), we speculated that an admixture-based approach may yield better results. To overcome the possible limitations of markers included on commonly used microarrays, we used the GenoChip, a dedicated genotyping array for population genetics [17] , which includes over 100,000 ancestral informative markers (AIMs). These autosomal AIMs were collected from the literature and captured using tools such as AimsFinder, which identifies the smallest number of markers sufficient to differentiate a pair of populations that are genetically distinct. AimsFinder was applied to private and public data sets for multiple populations, many of which were not studied before or searched for AIMs, and the recovered markers were included in the GenoChip. To overcome the methodological limitations, we developed an admixture-based Geographic Population Structure (GPS) method for predicting the biogeographical origin of worldwide individuals from resident populations. We demonstrated the performances of this method on three data sets and compared its results with those of SPA [12] . GPS outperformed SPA in all analyses, demonstrating the power of admixture-based tools to infer biogeography. GPS implementation The GPS method consists of two steps. In the first step, carried out once, we constructed a diverse panel of worldwide populations and analysed them using an unsupervised ADMIXTURE analysis. This analysis yielded allele frequencies for K hypothetical populations whose genotypes can be simulated to form putative ancestral populations. Next, from the data set of worldwide population, we constructed a smaller data set of reference populations that are both genetically diverse and have resided in their current geographical region for at least few centuries. These populations were next analysed in a supervised ADMIXTURE analysis that calculated their admixture proportions in relation to the putative ancestral populations ( Fig. 1 ). 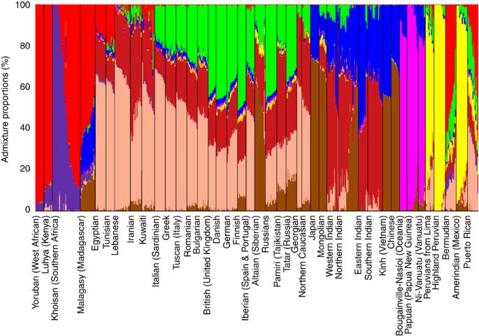Figure 1: Admixture analysis of worldwide populations and subpopulations. Admixture analysis was performed forK=9. For brevity, subpopulations were collapsed. Thexaxis represents individuals from populations sorted according to their reported ancestries. Each individual is represented by a vertical stacked column of colour-coded admixture proportions that reflects genetic contributions from putative ancestral populations. Figure 1: Admixture analysis of worldwide populations and subpopulations. Admixture analysis was performed for K =9. For brevity, subpopulations were collapsed. The x axis represents individuals from populations sorted according to their reported ancestries. Each individual is represented by a vertical stacked column of colour-coded admixture proportions that reflects genetic contributions from putative ancestral populations. Full size image Looking at the resulting graph, we found that all populations exhibit a certain amount of admixture, with Puerto Ricans and Bermudians exhibiting the highest diversity and Yoruba the least. We further found distinct substructure among geographically adjacent populations that decreased in similarity with distance, suggesting that populations can be localized based on their admixture patterns. To correlate the admixture patterns with geography, we calculated two distance matrices between all reference populations based on their mean admixture fractions (GEN) and their mean geographic distances (GEO) from each other. Using these distance matrices, we calculated the relationship between GEN and GEO (Equation 1). In the second step, GPS inferred the geographical coordinates of a sample of unknown origin by performing a supervised ADMIXTURE analysis for that sample with the putative ancestral populations. It then calculated the Euclidean distance between the sample’s admixture proportions and GEN. The shortest distance, representing the test sample’s deviation from its nearest reference population, was subsequently converted into geographical distance using the inferred relationships (Equation 1). The final position of the sample on the map was calculated by a linear combination of vectors, with the origin at the geographic centre of the best matching population weighted by the distances to M nearest reference population and further scaled to fit on a circle with a radius proportional to the geographical distance obtained by Equation 1 (see Calculating the bio-origin of a test sample in the Methods). Biogeographical prediction for worldwide individuals We applied GPS to approximately 600 worldwide individuals collected as part of the Genographic Project and the 1000 Genomes Project and genotyped on the GenoChip ( Supplementary Table 1 ). We included the highly heterogeneous populations of Kuwait [22] , Puerto Rico and Bermuda [23] , as well as communities from the same country, such as Peruvians from Lima and indigenous highland Peruvians. We tested the accuracy of GPS predictions using the leave-one-out procedure. The resulting figure bears a notable resemblance to the world’s geographic map ( Fig. 2 ). Individuals from the same geographic regions clustered together, and populations from different countries were largely distinguished. Assignment accuracy was determined for each individual based on whether the predicted geographical coordinates were within the political boundaries of the country and regional locations. GPS correctly assigned 83% of the individuals to their country of origin, and, when applicable, ~66% of them to their regional locations ( Fig. 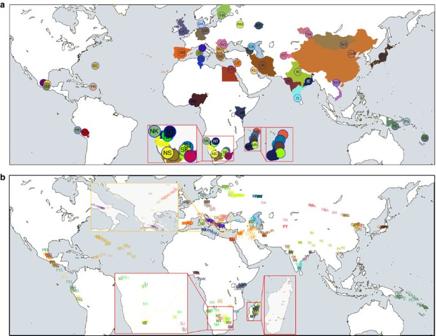Figure 2: Geographic origin of worldwide populations. (a) Small coloured circles with a matching colour to geographical regions represent the 54 reference points used for GPS predictions. Each circle represents a geographical point with longitude and latitude and a certain admixture proportion. The insets provide magnification for dense regions. (b) GPS individual assignment based on 54 points. Individual label and colour match their known region/state/country of origin using the following legend: BE (Bermudian), BU (Bulgarian), CHB (Chinese), DA (Danish), EG (Egyptian), FIN (Finnish), GO (Georgian), GR (German), GK (Greek), I-S/N/W/E (India, Southern/Northern/Western/Eastern), IR (Iranian), ID/TSI (Italy: Sardinian/Tuscan), JPT (Japanese), LWK (Kenya: Luhya), KU (Kuwaiti), LE (Lebanese), M-O/B/N/D/T (Madagascar: Antananarivo/Ambilobe/Manakara/Andilambe/Toliara), X-G/H/M (Mexico: Guanajuato/Hidalgo/Morelos), MG (Mongolian), N-S/K/H/T (Namibia: Southeastern/Kaokoveld/Hereroland/Tsumkwe), YRI (Yoruba from West African), P-C/N (Papuan: Papua New Guinea/Bougainville-Nasioi), PH/PEL (Peruvian: Highland/Lima), PR (Puerto Rican), RO (Romanian), CA (Northern Caucasian), R-M/T/A (Russians: Moscow/Tatarÿ/Altaian), S-J/U/S/K/ (RSA: Johannesburg/Underberg/Northern Cape/Free State), IBS (Iberian from Spain & Portugal), PT (Pamiri from Tajikistan), TU (Tunisian), UK (British from United Kingdom), VA (Vanuatu), KHV (Vietnam).Note: occasionally all samples of certain populations (for example, Vietnamese) were predicted to the same spot and thus appear as a single sample. 3 , Supplementary Table 2 ), with high sensitivity (0.75) and specificity (0.99). These results supported the known connection between admixture patterns and geographic origins in worldwide populations [5] , [6] , [7] , [8] . Figure 2: Geographic origin of worldwide populations. ( a ) Small coloured circles with a matching colour to geographical regions represent the 54 reference points used for GPS predictions. Each circle represents a geographical point with longitude and latitude and a certain admixture proportion. The insets provide magnification for dense regions. ( b ) GPS individual assignment based on 54 points. Individual label and colour match their known region/state/country of origin using the following legend: BE (Bermudian), BU (Bulgarian), CHB (Chinese), DA (Danish), EG (Egyptian), FIN (Finnish), GO (Georgian), GR (German), GK (Greek), I-S/N/W/E (India, Southern/Northern/Western/Eastern), IR (Iranian), ID/TSI (Italy: Sardinian/Tuscan), JPT (Japanese), LWK (Kenya: Luhya), KU (Kuwaiti), LE (Lebanese), M-O/B/N/D/T (Madagascar: Antananarivo/Ambilobe/Manakara/Andilambe/Toliara), X-G/H/M (Mexico: Guanajuato/Hidalgo/Morelos), MG (Mongolian), N-S/K/H/T (Namibia: Southeastern/Kaokoveld/Hereroland/Tsumkwe), YRI (Yoruba from West African), P-C/N (Papuan: Papua New Guinea/Bougainville-Nasioi), PH/PEL (Peruvian: Highland/Lima), PR (Puerto Rican), RO (Romanian), CA (Northern Caucasian), R-M/T/A (Russians: Moscow/Tatarÿ/Altaian), S-J/U/S/K/ (RSA: Johannesburg/Underberg/Northern Cape/Free State), IBS (Iberian from Spain & Portugal), PT (Pamiri from Tajikistan), TU (Tunisian), UK (British from United Kingdom), VA (Vanuatu), KHV (Vietnam). Note : occasionally all samples of certain populations (for example, Vietnamese) were predicted to the same spot and thus appear as a single sample. 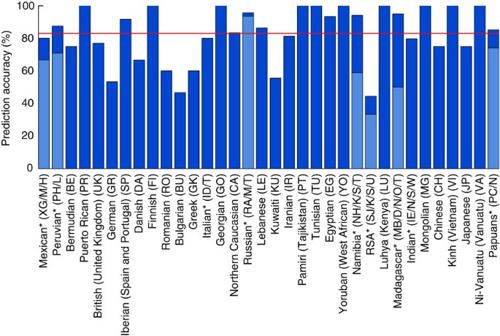Figure 3: Accuracy of assigning populations to their origin is coloured with dark blue for countries and light blue for regional locations. Populations for which regional data were available are marked with an asterisk. The average accuracy per population is shown in red and is calculated across populations given equal weights. Full size image Figure 3: Accuracy of assigning populations to their origin is coloured with dark blue for countries and light blue for regional locations. Populations for which regional data were available are marked with an asterisk. The average accuracy per population is shown in red and is calculated across populations given equal weights. Full size image In terms of distances from the point of true origin, GPS placed 50% of the samples within 87 km from the origin with 80 and 90% of them within 645 and 1,015 km from the origin, respectively. GPS further discerned geographically adjacent populations known to exhibit high genetic similarity, such as Greeks and Italians. The prediction accuracy was correlated with both countries’ area ( N =600, r =0.3, Student’s t -test P -value=0.03) and admixture diversity ( N =600, r =−0.34, Student’s t -test P -value=0.01). Individuals belonging to recently mixed populations, such as Kuwaitis and Bermudians, proved to be the most difficult to correctly predict, because their mixing was temporally brief and insufficient to generate a distinct regional admixture signature. As a result, such individuals are more likely to be placed within their original countries of origin, which is incorrect according to our scoring matric. For example, Kuwaiti individuals whose ancestors come from Saudi Arabia, Iran and other regions of the Arabian Peninsula [22] were predicted to come from these regions rather than their current state. To test GPS’s accuracy with individuals from populations that were not included in the reference population set, we conducted two analyses. We first repeated the previous analysis using the leave-one-out procedure at the population level. As expected, GPS accuracy decreased with 50% of worldwide individuals predicted to be 450 km away from their true origin. The predicted distance increased to 1,100 and 1,750 km for 80 and 90% of the individuals, respectively ( Fig. 4a ). Because GPS best localizes individuals surrounded by M genetically related populations, populations from island nations (for example, Japan and United Kingdom) or populations whose most related populations were under-represented in our reference population data set (for example, Peru and Russia) were most poorly predicted. Consequently, the median distances to the true origin were much smaller for individuals residing in Europe (250 km), Africa (300 km) and Asia (450 km) due to their being more commonly represented in the reference population data set compared with Native Americans and Oceanians. These results represent the upper limit of GPS’s accuracy when the specific population of the test individual is absent from the reference population data set. 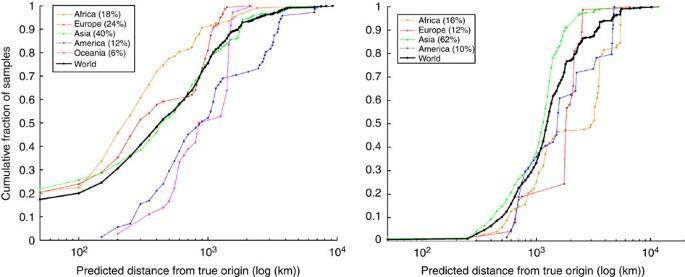Figure 4: Predicted distance from true origin for each individual using the leave-one-out procedure at the population level. Calculated for individuals of the Genographic (left) and the HGDP (right) data sets. Figure 4: Predicted distance from true origin for each individual using the leave-one-out procedure at the population level. Calculated for individuals of the Genographic (left) and the HGDP (right) data sets. Full size image Next, we analysed over 600 individuals from the Human Genome Diversity Panel (HGDP) whose subpopulations and populations reside in countries that are not covered by our reference population data set ( Supplementary Table 1 ). GPS’s accuracy further decreased with 50% of worldwide individuals predicted to be 1,250 km away from their true origin ( Fig. 4b , Supplementary Data 1 ). As before, geographically remote populations were less accurately predicted with a higher error for regions that were poorly represented in the reference population data set. For example, the Brazilian Surui were predicted to be located 4,800 km away from their true origin. This was not surprising because the closest population in the reference population data set resided in Central America. By contrast, remote European populations that reside on islands or along ocean shores and are not surrounded by other populations (for example, Orcadians and French) were predicted to be ~1,200 km from their true origin, due to the higher density of nearby populations in the reference population data set. The results were also affected by populations with a history of recent migrations, such as Bedouins, Druze [24] and the Pakistani Hazara, the latter being suspected of having some Mongolian ancestry [25] . Adding the HGDP populations to our reference population data set yielded similar results to those reported in Fig. 3 . Overall, these results illustrated the dependency of GPS on the density of the reference population data set and indicated that accuracy improves with the inclusion of additional populations residing in geographically distant or isolated regions. GPS applicability using a thinner marker set PC-based applications have long aspired to provide accurate results down to the level of an individual’s village. However, due to different factors such as cohort effects [26] , these solutions have been mostly ad hoc . In fact, PC solutions were shown to discern only populations of selected cohorts, such as Italian villagers [27] or Europeans [11] , [12] . When individuals of various ancestries are included in the cohort, the PCs are altered to the point where none of the individuals are correctly predicted to their country of origin or continental regions. To test the precision of GPS’s predictions given finer regional annotation, we assessed 243 Southeast Asians and Oceanians and 200 Sardinians from 10 villages (4–180 km apart) using subsets of 40,000 and 65,000 GenoChip markers, respectively. We first tested whether admixture frequencies calculated over a smaller set of GenoChip markers provided sufficient accuracy. For this assessment, we carried out a series of admixture analyses in a supervised mode for nine 1000 genomes worldwide populations using smaller sets of markers (95,000, 65,000 and 40,000) and compared the admixture proportions with those obtained using the complete marker set ( Fig. 5 ). We found small differences in the admixture proportions that slowly increased for smaller GenoChip marker sets. The largest observed difference (3%) for the smallest number of markers used in our analyses (40,000) was within the natural variation range of our populations and did not affect the assignment accuracy. We were thus able to supplement the reference population set with the newly tested populations. 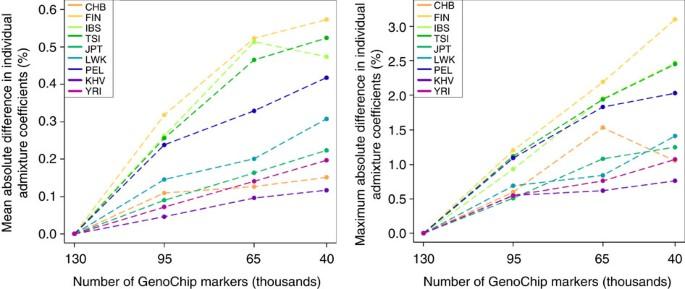Figure 5: Estimation of the bias in the admixture proportions of nine 1000 Genomes populations analysed over a reduced set of GenoChip markers. The mean (left) and maximum (right) absolute difference in individual admixture coefficients are shown. Figure 5: Estimation of the bias in the admixture proportions of nine 1000 Genomes populations analysed over a reduced set of GenoChip markers. The mean (left) and maximum (right) absolute difference in individual admixture coefficients are shown. Full size image Fine-scale biogeography down to home island Next applied to Southeast Asians and Oceanians ( Supplementary Table 3 , Supplementary Fig. 1 ), GPS’s prediction accuracy was stringently estimated as the individual assignment to the region occupied by one’s population or subpopulation. The prediction accuracy for Han Chinese (64%) and Japanese (88%) obtained here using ~40,000 markers was the same as that obtained in the complete data set, as expected ( Fig. 5 ). GPS’s assignment accuracy for the remaining Southeast Asian and Oceanian populations (87.5%) and subpopulations (77%) ( Fig. 6 ) was higher than that obtained for worldwide populations ( Fig. 3 ). These results reflect GPS’s greatest advantage compared with alternative methods. Unlike PCA and SPA whose accuracy is lost with the addition of samples of various ancestries [12] , GPS predictions increase in accuracy when provided a more comprehensive reference set. 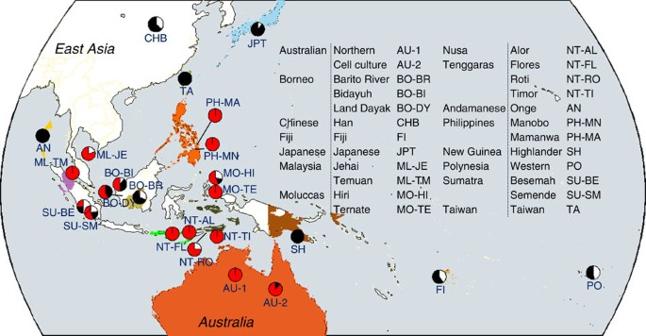Figure 6: Prediction accuracy for Southeast Asian and Oceanian subpopulations and populations. Pie charts depicts correct mapping at the subpopulation level (red), population level (black) and incorrect mapping (white). Figure 6: Prediction accuracy for Southeast Asian and Oceanian subpopulations and populations. Pie charts depicts correct mapping at the subpopulation level (red), population level (black) and incorrect mapping (white). Full size image A few populations stand out in that they are not reliably assigned to their region of origin ( Fig. 6 ). Polynesians and Fijians in particular are not well predicted and incur the highest misclassification rates (47 and 40%, respectively) mainly to Nusa Tenggara and the Moluccas Islands. These results are not surprising given two main issues. First, Polynesian populations, East Polynesian populations in particular, are not well represented in the large databases from which the GenoChip’s ancestry informative markers were ascertained [17] , so a likely ascertainment bias exists for Polynesia. The second issue relates to the complex settlement history of the Oceania region. Interestingly, this aspect of population history is clearly reflected in the results produced. The component identified in the admixture analysis ( Supplementary Figure 1 ) as representing Oceania (pink) most likely represents the early migrants into the region some 50,000 years ago. This component is dominant in populations from New Guinea and Australia, which were joined together, making up the ancient landmass of Sahul, until approximately 11,000 years ago when they became separated due to rising sea levels. This Oceanic signature is also seen in Island Southeast Asia, such as Nusa Tenggara and the Moluccas, which indicates the likely pathway taken to Sahul. The Remote Oceanic settlement, represented here by Fiji and Polynesia, is much more recent and has been associated with the Neolithic expansion of peoples out of East Asia, through Island Southeast Asia and ultimately through Near Oceania and the rest of the Pacific including Polynesia. The first people to arrive in Remote Oceania (the region east of the Solomon Islands) did so only about 3,000 years ago and are associated with the expansion of the Lapita cultural complex as far east as Fiji, Samoa and Tonga, on the edge of the Polynesian Triangle. Mitochondrial DNA and Y chromosomal data from Remote Oceanic populations, Polynesians in particular, indicate mixed ancestry [28] . MtDNA suggests primarily Island Southeast Asian ancestry for Remote Oceania, indicated by high frequencies of mtDNA haplogroup B4a1a and descendent lineages, with some Near Oceanic contributions (identified by haplotypes belonging to haplogroups P and Q). Y chromosome studies, however, show a stronger Near Oceanic component in Polynesian ancestry, with some Southeast Asian contribution [29] . Genome-wide studies are consistent with this mixed ancestry for Polynesian, Remote Oceanic and some Near Oceanic populations [30] . Our findings, therefore, represent the heterogeneity of Remote Oceanian populations due to their long history of expansions and settlements, which is reflected by their complex population structure ( Supplementary Fig. 1 ) and GPS predictions ( Fig. 6 ). Fine-scale biogeography down to home village The island of Sardinia (24,090 km 2 ) was first settled 14,000 years ago and experienced a complex demographic history that includes low effective sizes due to plagues and wars and scant matrimonial movement, which accentuated stochastic effects. Interestingly, Sardinians have been described both as a genetic isolate with endogamy peaking in the central-southern and mountain areas with little internal mobility [31] and a heterogeneous population when microareas or close single village are considered [32] , [33] , [34] . Applied to Sardinian villagers ( Supplementary Fig. 2 ), GPS correctly placed a quarter of the Sardinians in their village, as well as half within 15 km and 90% of individuals within 100 km of their homes ( Fig. 7 , Supplementary Fig. 3 ). As expected from the high percentages of matrilocal marriages [35] and residence [36] , [37] common to Sardinia, the locations of females were better predicted than those of males, with 30% placed in their exact village of origin compared with 10% of the males. 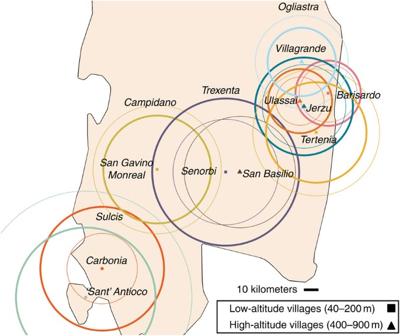Figure 7: The geographical location of the examined Sardinian villages. The mean predicted distances (km) from the village of origin are marked by bold (females) and plain (males) circles. Figure 7: The geographical location of the examined Sardinian villages. The mean predicted distances (km) from the village of origin are marked by bold (females) and plain (males) circles. Full size image Our findings revealed the Sardinians to have a genetic microheterogeneous structure affected both by altitude and physical location. The prediction accuracy as the distance to the village of origin ( Supplementary Fig. 3 ) are detailed in Supplementary Table 4 . The correlations between altitude and the distance from the village of origin are shown in Supplementary Table 5 . The average predicted distances from the villages roughly corresponded to Sardinian subregions ( Fig. 7 ). Unsurprisingly, the more precise positioning refers to individuals coming from Ogliastra (east Sardinia), since this area is characterized both by high altitude, high endogamy and relative cultural isolation, whereas populations from the western shores are considered to be more admixed. We found a significantly negative correlation between altitude and the predicted distance to villages for males ( N (coastal)=96, r (coastal)=−0.21, Student’s t -test P -value(coastal)=0.019; N (coastal)=27, r (inland)=−0.38, Student’s t -test P -value(inland)=0.024). The results for females were marginally significant for all villages ( N =126, r =−0.14, Student’s t -test P =0.06) and inland villages ( N =29, r =−0.27, Student’s t -test P =0.08), but not for coastal villages ( N =97, r =−0.1, Student’s t -test P =0.14). These results are expected from the high proportion of endogamy (64.1% in plain, 82.8% in mountains) that are correlated with the rise of altitude [35] . This correlation was particularly high in inland compared with coastal villages. Our results not only fit with the genetic and demographic characteristics of Sardinians but also resolve conflicting findings due to the matrilocal matrimonial structure [36] , [38] , [39] , [40] . Finally, because GPS carries a sample-independent analysis, predictions for worldwide individuals were largely identical to those previously reported ( Fig. 3 ) in both analyses. Comparing the performances of GPS with SPA The SPA tool explicitly models the spatial distribution of each SNP by assigning an allele frequency as a continuous function in geographic space [12] . SPA can model the spatial structure over a sphere to predict the spatial structure of worldwide populations and was designed to operate in several modes. In one mode, when the geographic origins of the individuals are known or when the geographic origins of some individuals are known, they can be used as training set. Using the later approach, Yang et al . [12] trained the SPA model on 90% of the individuals to predict the locations of the remaining 10%. SPA was reported to predict the geographic origins of individuals of mixed ancestry, which cannot be done with PCA [12] . When analysing a Europeans-only data set, SPA was successful in assigning close to 50% of the individuals to their correct country of origin. However, when worldwide individuals were analysed, SPA distorted the distances between continents and failed to assign even a single individual to his home country ( Fig. 8a ), with Melanesians being misclassified as Indians [12] being the most obvious example. 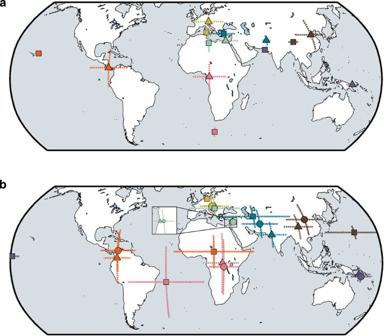Figure 8: A comparison of SPA and GPS prediction accuracy for continental regions. The mean longitude and latitude for each population were calculated by averaging individual spatial assignments (N=596). After assigning populations to continental regions, the mean and s.d. were calculated based on the predicted coordinates for each region. Dashed lines mark s.d. (a) SPA prediction accuracy for continental regions obtained from Yanget al.12results (theirsupplementary Table 112). The mean coordinates are marked with a triangle (expected) and square (Predicted by SPA). (b) Comparing the results for worldwide populations analysed here for SPA (square), GPS (circle) and for the real coordinates (triangle). Figure 8: A comparison of SPA and GPS prediction accuracy for continental regions. The mean longitude and latitude for each population were calculated by averaging individual spatial assignments ( N =596). After assigning populations to continental regions, the mean and s.d. were calculated based on the predicted coordinates for each region. Dashed lines mark s.d. ( a ) SPA prediction accuracy for continental regions obtained from Yang et al . [12] results (their supplementary Table 1 [12] ). The mean coordinates are marked with a triangle (expected) and square (Predicted by SPA). ( b ) Comparing the results for worldwide populations analysed here for SPA (square), GPS (circle) and for the real coordinates (triangle). Full size image We compared the accuracy of GPS with that of SPA by providing SPA with favourable conditions to its operation. We used the more rigorous application involving a training data set and ran SPA in two steps, as described by Yang et al . [12] . First, we provided SPA with the genotype file of worldwide populations (596 individuals, 127,361 SNPs) with their complete geographic locations ( Supplementary Table 2 ) without any missing data. When executed, SPA produced the model file that would be later used to predict the geographical locations. Next, we provided SPA with the model file and the same genotype file. Because of the absence of missing geographical coordinates, SPA was expected to yield geographic coordinates that closely resemble those it received in the first step. However, SPA failed to assign 98% of individuals to their countries and placed most individuals in oceans or in the wrong continental region ( Fig. 8b ). By comparison, GPS was used in the leave-one-out individual mode, in which the geographic coordinates of the populations in the reference population data set were recalculated without the test individual. GPS accurately assigned nearly all individuals to their continental regions, countries and regional locations with a high degree of accuracy. We tested SPA with four additional data sets and calculated the assignment accuracy for each one. When providing SPA with the combined data set of worldwide individuals and Southeast Asian and Oceanian individuals (~40,000 SNPs) with their complete geographical coordinates ( Supplementary Table 3 ), we obtained a similar assignment accuracy of 2% for the worldwide individuals, although with different coordinates and an assignment accuracy of 1.5% for the remaining individuals. When testing only Southeast Asian and Oceanian individuals, the assignment accuracy was 4.8%. Unfortunately, we were unable to estimate the prediction accuracy for about 20% of these samples because SPA’s results (e.g., Latitude=−2, Longitude=256) exceeded those of a three-dimensional sphere. Finally, we calculated the assignment accuracy for worldwide individual and Sardinian individuals (~65,000 SNPs), again by providing complete geographical data ( Supplementary Table 4 ). SPA coordinates for worldwide individuals varied from our previous analyses, being accurate for three individuals (0.5%) but completely inaccurate (0%) for Sardinians whether they were tested with the worldwide individuals or separately. We suspect that the inaccuracy of SPA predictions in the tested mode of operation results from the predictions for test individuals being affected by other individuals in the cohort. As such, it suffers from the same limitations as PCA when analysing a diverse cohort. Even if a single individual from a different continent is included in the data set, SPA’s accuracy drops to 0%. In other words, for SPA to correctly assign every other European individual to his country, the individuals need to be a priori confirmed as Europeans, which makes SPA impractical. A comparison of the runtime and CPU timings was done on a Linux machine (x86 64) with an Intel(R) Xeon(R) E5430 processor 2.66 GHz CPU and 8 GB memory. The SPA runtime (wall time) was well over 3 h, compared with 6 min for GPS, including the initial step of calculating admixture proportions using ADMIXTURE. We present a solution to one of the most challenging problems of biogeography: localizing individuals based on their genetic data. Our solution consists of analysing populations genotyped over a relatively small set of AIMs and applying an admixture-based GPS method to predict their origin. We have shown that our approach can predict the geographical origin of worldwide individuals from single resident populations down to the level of island and home village and is more accurate than SPA. Some of the limitations of SPA and PCA for inferring ancestral origin have been previously noted [12] , [16] . A major limitation of these methods for biogeography is their specificity to relatively homogeneous populations, such as Europeans, and their susceptibility to biases caused by populations of different ancestry, as is the case with real-life data. SPA’s assignment accuracy ranged between 0 and 4.8% with predictions varying over different runs for the same individuals. By averaging over all data sets, we estimated SPA’s assignment accuracy to be 1.5%. These results contradict those reported by Yang et al . [12] for European populations, whose estimation is based on a European-only data set. However, when worldwide populations were used, the results of Yang et al . [12] ( Fig. 8a ) are in agreement with ours ( Fig. 8b ). By contrast, GPS is a sample-independent method that relies on a fixed set of reference populations to predict the individual’s geographical origin irrespective of the tested cohort. We have shown that GPS successfully localized 83% of worldwide individuals to their country of origin and that its accuracy increased with the addition of more localized and well-annotated populations such as Southeast Asians, Oceanians and Sardinians. The advantage of using reference populations becomes apparent when analysing migratory populations that have relocated yet maintained endogamy. Such populations present a formidable concern to biogeographic methods that rely on the relationships between geography and genetics [5] , [6] , [7] , [8] . In theory, SPA would yield biased results if the immigrant population with its current geographical location would be used for training or be included in the test cohort with populations located nearby its modern-day region. Unfortunately, the low accuracy of SPA prevents us from demonstrating this effect, although it was noted for a similar approach, PCA [12] , [16] . GPS addresses this concern by using a reference population set that excludes such populations and by adopting a sample-independent approach. The success of this approach was demonstrated with the Kuwaitis, who comprise an amalgam of populations that were predicted to their former origin ( Fig. 2 ). We have further demonstrated the accuracy of our approach when using only 40,000 markers, making GPS applicable to genetic data genotyped on the most common microarrays. Overall, GPS’s accuracy, high sensitivity and specificity, along with its memory efficiency and high speed, make it a powerful tool for biogeography and related scientific fields. Given these successes, GPS has other potential applications. For example, in genealogical research, it could help adoptees find their home region, while, in forensic research, it could improve the assignment of ethnic (geographic) ancestry to DNA evidence. Although common wisdom in genetics is that ‘more is better,’ we demonstrate that only tens of thousands of AIMs are sufficient to accurately infer biogeography down to the home village, provided that the appropriate samples are available in the reference population data set. We emphasize that GPS may not necessarily yield the most recent region of residency for populations that experienced recent admixture or have recently migrated and maintained a certain degree of endogamy, but rather a historical residency. Therefore, the region of origin can be intuitively interpreted as where the last major admixture took place at the population level since the establishment of the reference populations in their provided geographical location. We envision that, with time, biogeographical applications will become enhanced for more worldwide communities due to the addition of populations to the reference panel. Therefore, our results should be considered a lower bound to the full potential of GPS for biogeography. We hope that our study will promote new thinking about how population size, genetic diversity and environment have shaped human population structure. Sample collection and genotyping Genographic sample collection was conducted according to the ethical protocol of The Genographic Project ( https://genographic.nationalgeographic.com/wp-content/uploads/2012/07/Geno2.0_Ethical-Framework.pdf ), with oversight provided by the University of Pennsylvania and regional IRBs (specified in the original reports from which data analyzed in this study were taken). IRBs were obtained for new collections in Italy, UK, Denmark, Greece, Germany and Romania (sample and data collection were undertaken with approval from the IRB, Comitè Ètic d’Investigació Clínica—Institut Municipal d’Assistència Sanitària (CEIC-IMAS) in Barcelona (2006/2600/I)); Peru (sample and data collection were undertaken with approval from the local IRB at Universidad San Martin de Porres, Lima, Peru; Federal Wide Assurance (FWA) for International Protection of Human Subject 0001532; US Health and Human Services (HHS) International Review Board IRB0000325); Puerto Rico (sample and data collection were undertaken with approval from the University of Pennsylvania IRB #8 and the support of Liga Guakia Taina-Ke); Mexico (sample and data collection were undertaken with approval from the University of Pennsylvania IRB #8, the Centro de Investigación y de Estudios Avanzados del Instituto Politécnico Nacional (CINVESTAV-IPN), and the Comision Nacional para el Desarrollo de los Pueblas Indigenas (CDI)); Egypt, Iran, Kuwait, Lebanon and Tunisia (the sample and data collection protocol were originally approved by the IRB committee of the Lebanese American University); North Eurasia (North Eurasia sample and data collection were undertaken with approval from the Ethical Committee of the Research Centre for Medical Genetics RAMS and the Academic Council of the same Research Centre); India (the sample and data collection protocol were originally approved by IRB of Madurai Kamaraj University, Madurai, India). Approval for further sampling, studies and collaborations have been obtained from IRB of Chettinad Academy of Research & Education, Kelampakka, India. Thirteen of the 65 samples studied from Tamil Nadu have already been investigated for NRY chromosomes [41] ( Supplementary Table S3 [41] )). In South Africa, sample and data collection was undertaken with approval from the Human Research Ethics Committee (University of the Witwatersrand, South Africa, Protocol Number M120151) under the auspices of grants from the South African Medical Research Council to HS. Data for three Italian samples were undertaken with approval of the Ethics Committee for Clinical trials of the University of Pisa (N. 3803). In Oceanian, the Nasioi samples were obtained from the HGDP-CEPH repository, whereas the Papuan and Vanuatu samples were previously published [42] , [43] . All participants provided written informed consent for the use of their DNA in genetic studies. Samples were collected under the same criteria requiring unrelated individuals with four grandparents from their population affiliation and geographic region of origin ( Supplementary Table 3 ). We also genotyped nine populations from the 1000 Genomes Project, including Mexican-Americans, African-Americans, Peruvians from Lima, Finns, Yoruba, Luhya from Kenya, Han Chinese, Japanese and Kinh from Vietnam. Overall, we sampled 615 unrelated individuals representing 98 worldwide populations and subpopulations with ~15 samples per population. Samples were genotyped on the GenoChip array, an Illumina HD iSelect genotyping bead array dedicated solely for genetic anthropology and lacking medically relevant markers. The GenoChip includes nearly 150,000 highly informative Y-chromosomal, mitochondrial, autosomal and X-chromosomal markers, of which only autosomal markers (~130,000) were used. We obtained the HGDP data set available at ftp://ftp.cephb.fr/hgdp supp10/ [44] and the geographical coordinates for each sample [45] . From the 828 samples reported to include no outliers using the filtering procedure used by Patterson and colleagues [44] , we excluded 201 samples for which no clear geographical origin was described or that their populations were already included in our reference population panel ( Supplementary Data 1 ). Because of the size of China and the high representation of Chinese populations in the HGDP data set, we excluded only the Han Chinese. Assessing data quality Data quality was achieved by applying two criteria to the SNP data. The first was low missingness rate (<5%), calculated as the average number of null genotypes over all samples in a population. In addition, individuals that exhibit distinct admixture proportions compared with samples of the same populations were considered outliers and omitted. Overall, we omitted 2,423 SNPs and seven Genographic samples from the analysis. Generating putative ancestral populations To infer the putative ancestral populations, we applied ADMIXTURE [46] in an unsupervised mode to the filtered data set. This analysis uses a maximum likelihood approach to determine the admixture proportions of the individuals in question assuming they emerged from K hypothetical populations. We speculated that our method will be the most accurate when populations have uniform admixture assignments. In choosing the value of K that seemed to best satisfy this condition, we experimented with different K s ranging from 6 to 12. We identified a substructure at K =10 in which populations appeared homogeneous in their admixture composition. Higher values of K yielded noise that appeared as ancestry shared by very few individuals within the same populations. ADMIXTURE outputs the speculated allele frequencies of each SNP for each hypothetical population. Using these data, we simulated 15 samples for each hypothetical population and plotted them in a PCA analysis with the Genographic populations. We observed that two hypothetical populations were markedly close to one another, suggesting they share the same ancestry and eliminated one of them to avoid redundancy. The remaining nine populations were considered the putative ancestral populations and were used in all further analyses. Creating a reference population data set To infer the geographical coordinates (latitude and longitude) of an individual given his K admixture frequencies, GPS requires a reference population set of N populations with both K admixture frequencies and two geographical coordinates (longitude and latitude). We omitted four populations for which we had no clear geographical data, were recently admixed populations or had a recent migratory history and did not maintain strict endogamy (African and Mexican-Americans, Brahmin Indians and Romanian Gypsies), as they were reported to deviate from the established relationship between genetic and geographic distances [7] and cannot be expected to be predicted to their present day origin correctly. The final data set consisted of 596 unrelated individuals representing 94 worldwide populations and subpopulations with an average of 17 individuals per population and at least two individuals per subpopulation ( Supplementary Table 3 ). These populations were considered hereafter as reference populations, since their admixture frequencies were calculated by applying ADMIXTURE in a supervised mode with the nine putative ancestral populations ( Fig. 1 ). Although few populations included detailed annotation for subpopulations within the parental populations (for example, Tuscany and Sardinian Italians), such annotation was unavailable for most populations, even though they exhibited fragmented subpopulation structure. This heterogeneity is expected given the young age of some of the populations. For example, using an internal data set, we were able to verify that the observed substructure among Germans was due to individuals from both West and East Germany. A combination of several criteria was employed to determine the number of subpopulations present within the study populations. Let N a denote the number of samples per population a ; if N a was less than three, the population was left unchanged. For other populations, we used k -means clustering routine in R . Let X ij be the admixture proportion of individual i in component j . For each population, we ran k -means clustering for k ∈ [2,4], using N a × 9 matrix of admixture proportions ( X ij ) as input. At each iteration, we calculated the ratio of the sum of squares between groups and the total sum of squares. If this ratio was >0.9, then we accepted the k -component model. Since k -means clustering cannot be implemented for k =1, to decide between two clusters or a possible single cluster, we also calculated Kullback-Leibler distance (KLD) between the k =2 and k =1 models. If the KLD <0.1 and the ratio of the sum of squares between groups and the total sum of squares for two-component model is above 0.9, then the k =1 model was selected because, in such cases, there are no subgroups in the population. Of the 216 subclusters detected, we excluded all the subclusters that contained only one individual. Overall, we included 146 subpopulations in our reference population set and determined the Mean admixture coefficients for each subpopulation. Calculating the relationship between admixture and geography GPS implements a genetic clustering approach that uses the relationship between admixture and geography to predict geograpical locations. To correlate the admixture patterns with geography, we calculated two distance matrices between all reference populations based on their mean admixture fractions (GEN) and their mean geographic distances (GEO) from each other. Next, given a matrix GEN of nine admixture coefficients for N populations and a matrix GEO with two geographical coordinates of latitude and longitude for N populations, we calculated the Euclidean distances between all the populations within the GEN and GEO data sets. For the GEN data set, the distances were computed as , where X and Y denote individuals with known origins; X k and Y k , k =1,…, K represent admixture proportions for the analysed individuals. For the GEN data set, the genetic distances Δ GEO ( X , Y ) between two individuals with known latitude and longitude were calculated using the Haversine formula [47] : , where R is the radius of Earth (for simplicity assumed to be equal to 3,959 miles), δ lat = lat 2 − lat 1 , and δ lon = lon 2 − lon 1 . The relationship between Δ GEO and Δ GEN was approximately linear for distances below 5,000 miles ( Fig. 9 ). 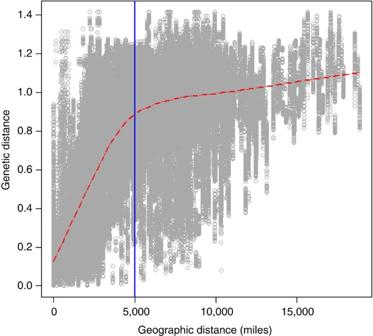Figure 9: Geographic versus genetic distances plotted for every two worldwide individuals. A loess distribution fitting is shown in red line with blue bar marking the limit of the linear fitting. Figure 9: Geographic versus genetic distances plotted for every two worldwide individuals. A loess distribution fitting is shown in red line with blue bar marking the limit of the linear fitting. Full size image Using linear regression and filtering out geographic distances above 4,000 miles, we determined intercept (β) and slope (α) for the relationship between genetic (Δ GEN ) and geographic distances (Δ GEO ): The relationship between genetics and geography obtained using Equation 1 varied across continents. Although this may be a true effect, it is more likely to be an artefact due to low sample density for non-European populations. Because we analyze geographically local population structure, we applied the intercept and slope calculated for Europeans as β=38.7 and α=2,523 for non-European populations for which sampling density was lower and thus local regression is less reliable. This regression equation should be refined with the addition of new population samples. Calculating the biogeographical origin of a test sample Given nine admixture proportions for a sample of unknown geographic origin obtained using ADMIXTURE’s supervised approach with the nine putative ancestral populations, we calculated the Euclidean distance between its admixture proportions and the N reference populations (GEN). All reference populations were sorted in an ascending order according to their genetic distance from the sample. The smallest distance represented the sample’s deviation from the best matching population. This distance in genetic space was converted into geographic distance using Equation 1. The contribution of other reference populations m =2… N to the samples’ genetic make-up is represented using the weight , where is the distance to the m th reference population. To refine the positioning of the sample, we used M closest reference populations (default value is M =10). Because GPS relies on the linear relationship between genetic and geographic coordinates, which holds for populations that are less than 4,000 miles apart, the value of parameter M depends on the density of the reference population data set. A data set with few populations that are geographically sparse would require a smaller M . We determined the value of M empirically by increasing the number of nearest populations ( M ) and observing changes of geographic coordinates. We found that the addition of extra populations after M reaches 10 does not significantly affect the prediction. The predicted position of the sample on the map is computed using Equation 2 below which is a linear combination of vectors with the origin at the geographic centre of the best matching population ( Position best ), weighted by w and scaled to fit on the circle with a radius : where Position ( m ) is the geographic center of the m th population, and γ denotes the scaling coefficient to ensure that predicted position fits on the circle with radius , equals to Intuitively, the predicted position of a test sample can be thought of as being determined by M nearest reference populations, each ‘pulling’ in its direction with a strength proportional to its genetic distance from the test sample. The shorter the genetic distance to the reference population, the smaller is the assumed genetic difference and the higher is the pull. We thus ‘anchored’ the centre at the nearest reference population and represented the influence of the remaining M -1 nearest reference populations using a linear combination of two-dimensional vectors with the length of each vector inversely proportional to the genetic distance between the test sample and the reference populations. The direction of these vectors is calculated using the difference between the coordinate of the best matching reference population to those of all other M -1 nearest reference populations. Therefore, GPS best predicts populations that are geographically surrounded by the reference populations. Estimating the accuracy of GPS Different measures of assignment accuracy have been proposed in published studies. For example, Novembre et al . [11] estimated the distance from the country of origins, whereas Yang et al . [12] used a more stringent criterion of defining success as assigning individuals to their country of origin. To compare GPS’s accuracy to those of SPA [12] , we adopted the more stringent criteria of Yang et al . [12] . Assignment accuracy for subpopulations was based on the political and municipal boundaries of the regional locations. To estimate GPS’s assignment accuracy, we utilized the ‘leave-one-out’ approach at the individual level. In brief, we excluded each reference individual from the data set, recalculated the mean admixture proportions of its reference population, predicted its biogeography, tested whether it is within the geographic regions of the reported origin and then computed the mean accuracy per population. More specifically, we assumed that our individual is the j th sample from the i th population that consists of n i individuals. For all populations, excluding the individual in question, the average admixture proportion and geographical coordinates were calculated as: where θ m,s is the parameter vector for the s th individual from the m th population, and n m is the size of the m th population. For the i th population the adjusted average will be Last, we computed the best-matching population for each ‘left-out’ individual and calculated the proportion of individuals that are mapped to the correct continental region, country and, if applicable, regional locations for each population. In a similar manner, we utilized the ‘leave-one-out’ approach at the population level. That is, we excluded one population at a time from the reference population set, predicting the biogeography of the samples of that population, calculating their predicted distance from the true origin and computing the mean accuracy per continental populations and all samples. To calculate GPS accuracy for the HGDP samples, we followed the procedure described in the above section and calculated the distances from the predicted to the true origin of each individual. To evaluate the sensitivity and specificity per population, we counted the number of samples of the population in the country of interest predicted to their true country as true positives, the number of samples from other countries assigned to the country of interest as false positives, the number of samples from the country of interest assigned to other countries as false negatives and finally the number of samples from other countries that were not assigned to the country of interest as true negatives. Applying GPS to Southeast Asia and Oceania populations A data set of 243 individuals genotyped over 350,000 markers was obtained with permission from Reich et al . [48] Admixture proportions of individuals were calculated by applying ADMIXTURE in a supervised mode with the nine putative ancestral populations on the ~40,000 autosomal markers that overlapped with the GenoChip markers ( Supplementary Figure 1 ). The mean admixture proportions of these populations and their geographical coordinates were added to our reference population data set. In addition, we analysed 88 Han Chinese (CHB) and 87 Japanese (JPT) populations from this data set, even though they were already included in the worldwide data set and calculated their admixture in a similar manner. The admixture proportions of the CHB and JPT were similar to those reported in Fig. 1 . Applying GPS to Sardinian populations Genotype data of 290 Sardinian individuals from 28 villages genotyped on an Affymetrix array with nearly 700,000 markers was obtained with permission from Piras et al . [40] Each individual had four grandparents living in the same village. Genotype data were from four subregions: Ogliastra, Trexenta, Sulcis and Campidano. In particular, Ogliastra is a mountainous area characterized as a genetic isolate differentiated from the rest of the island and constituted by different villages with high endogamy, low immigration and high genetic differentiation. Conflicting results from studies that have investigated the internal genetic structure of different macroareas [38] , [39] , [40] suggest that the internal heterogeneity among the macroareas is limited to particular areas. After filtering out villages with insufficient data, ten villages with 249 individuals remained ( Supplementary Table 4 ). We obtained admixture proportions for the remaining individuals by applying ADMIXTURE in a supervised mode with the nine putative ancestral populations on the ~65,000 autosomal markers that overlapped GenoChip’s markers ( Supplementary Fig. 2 ). The mean admixture frequencies of these ten Sardinian populations and their geographical coordinates were added to our reference population data set. GPS availability Data, GPS R code and GPS on-line calculator are available on http://chcb.saban-chla.usc.edu/gps/ . GPS code can be found in the Supplementary Note . SPA’s code for Linux was obtained from the author’s website: http://genetics.cs.ucla.edu/spa/binary/linux.zip . How to cite this article: Elhaik, E. et al . Geographic population structure analysis of worldwide human populations infers their biogeographical origins. Nat. Commun. 5:3513 doi: 10.1038/ncomms4513 (2014).